Suppression of adult neurogenesis impairs population coding of similar contexts in hippocampal CA3 region Different places may share common features, but are coded by distinct populations of CA3 neurons in the hippocampus. Here we show that chemical or genetic suppression of adult neurogenesis in the hippocampus impairs this population-based coding of similar (but not dissimilar) contexts. These data provide a neural basis for impaired spatial discrimination following ablation of adult neurogenesis, and support the proposal that adult neurogenesis regulates the efficiency of a pattern separation process in the hippocampus. The ability to distinguish between different places is an essential feature of the hippocampal episodic memory system [1] . Computational models initially proposed that this is mediated by a pattern separation process within the hippocampal dentate gyrus (DG)-CA3 circuit [2] , and recent electrophysiological recording studies in rodents provide direct support for this view [3] , [4] , [5] . The DG and CA3 appear to code context changes differently. In the DG, context shifts produce changes in firing rate of the same population of active neurons (that is, a rate code), whereas the same context shifts alter the populations of cells firing in CA3 (that is, a population code) [3] , [4] . This CA3 population-based code of distinct environments may also be revealed using activity-dependent gene mapping of neuronal activation following exposure to the same versus different contexts [6] . As new neurons are added to the DG throughout adulthood [7] , this putative process of pattern separation occurs in a continuously evolving DG-CA3 circuit. Therefore, here we ask whether adult neurogenesis in the DG modulates the efficiency of context coding in the downstream CA3 region. To visualize the population code in CA3 we used a cellular imaging approach that takes advantage of the transcriptional time course of the activity-regulated cytoskeleton-associated protein ( arc ) (also known as Arg3.1) [8] . Following neuronal activation, arc mRNA is rapidly induced in the nucleus (within 5 min), but subsequently shuttled to the cytoplasm (within 25 min). Therefore, the localization of arc RNA (either in the nucleus, cytoplasm or both) identifies neuronal ensembles activated by separate context exposures. Accordingly, we used this technique to examine the effects of suppressing adult neurogenesis on activation of populations of CA3 neurons following exposure to the same, similar or dissimilar contexts. We found that suppression of adult neurogenesis impairs CA3 population coding of similar contexts. Chemical reduction of neurogenesis impairs population coding We first used a chemical approach to suppress adult neurogenesis (see Supplementary Methods ). Wild-type (WT) mice were treated with the DNA-alkylating agent Temozolomide (TMZ) or vehicle (VEH) for 4 weeks. Consistent with previous studies [9] , we observed that TMZ treatment suppressed adult neurogenesis, reflected by both a reduction in the number of DG cells expressing the proliferation marker, Ki67, and cells expressing the immature neuronal marker, NeuroD ( Fig. 1a ). Importantly, TMZ did not appear to compromise immune function (leukocyte recovery), alter general behaviour or lead to weight loss ( Supplementary Fig. S1 ). Next, separate cohorts of VEH- and TMZ-treated mice were habituated to two similar contexts (A, triangular-shaped; B, square-shaped), located in the same room. Twenty-four hours later, mice were either exposed to context A twice (AA condition), context A then B (AB condition) or context A then a novel, dissimilar context (C, rectangular-shaped and located in a different room; see Supplementary Fig. S2 ) (AC condition). Context exposures were separated by 20 min and brains were removed immediately after the second exposure and processed for arc fluorescent in situ hybridization to identify populations of CA3 neurons activated by the first (cytoplasmic arc ) and/or second (intranuclear arc ) context exposure ( Fig. 1c and Supplementary Fig. S3 ). 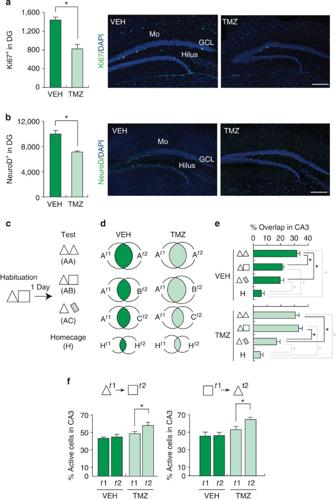Figure 1: Chemical Suppression of adult neurogenesis impairs coding of similar contexts. (a) Ki67+and (b) NeuroD+staining was reduced in TMZ-treated (n=4) compared with VEH-treated (n=4) mice, indicating that TMZ treatment reduced proliferation (t6=5.36,P<0.01) and the number of immature neurons (t6=5.09,P<0.01) in the DG, respectively. Scale, 200 μm. Mo, molecular layer, GCL, granule cell layer. (c) Experimental design. TMZ-treated and VEH-treated mice were habituated to contexts A (triangle) and B (square), and then tested in context A consecutively (AA; VEH,n=8, TMZ,n=8), context A then context B (AB; VEH,n=9, TMZ,n=10) or context A then context C (AC; VEH,n=10, TMZ,n=8) or home cage (H; VEH,n=4, TMZ,n=5). (d) Venn diagrams indicating populations of CA3 cells activated either by first (t1), second (t2) or both (overlap, shaded) context exposures, as reflected byarcexpression (context exposures>home cage,t-tests,P<0.05). (e) Percent of CA3 cells activated by both context exposures in VEH- versus TMZ-treated mice (Treatment × Context interaction,F3,54=4.43,P<0.01; Tukeypost-hoctests, *P<0.05). (f) Percent of CA3 cells activated on second (t2) versus first (t1) context exposure in VEH-treated (n=7) versus TMZ-treated (n=7) mice (t2>t1in AB [t9=3.11,P<0.05] and BA [t6=2.41,P=0.05] only in TMZ-treated mice). In these graphs, error bars represent s.e.m., and significantly different contrasts are marked by * (whereP<0.05). Figure 1: Chemical Suppression of adult neurogenesis impairs coding of similar contexts. ( a ) Ki67 + and ( b ) NeuroD + staining was reduced in TMZ-treated ( n =4) compared with VEH-treated ( n =4) mice, indicating that TMZ treatment reduced proliferation ( t 6 =5.36, P <0.01) and the number of immature neurons ( t 6 =5.09, P <0.01) in the DG, respectively. Scale, 200 μm. Mo, molecular layer, GCL, granule cell layer. ( c ) Experimental design. TMZ-treated and VEH-treated mice were habituated to contexts A (triangle) and B (square), and then tested in context A consecutively (AA; VEH, n =8, TMZ, n =8), context A then context B (AB; VEH, n =9, TMZ, n =10) or context A then context C (AC; VEH, n =10, TMZ, n =8) or home cage (H; VEH, n =4, TMZ, n =5). ( d ) Venn diagrams indicating populations of CA3 cells activated either by first ( t 1 ), second ( t 2 ) or both (overlap, shaded) context exposures, as reflected by arc expression (context exposures>home cage, t -tests, P <0.05). ( e ) Percent of CA3 cells activated by both context exposures in VEH- versus TMZ-treated mice (Treatment × Context interaction, F 3,54 =4.43, P <0.01; Tukey post-hoc tests, * P <0.05). ( f ) Percent of CA3 cells activated on second ( t 2 ) versus first ( t 1 ) context exposure in VEH-treated ( n =7) versus TMZ-treated ( n =7) mice ( t 2 > t 1 in AB [ t 9 =3.11, P <0.05] and BA [ t 6 =2.41, P =0.05] only in TMZ-treated mice). In these graphs, error bars represent s.e.m., and significantly different contrasts are marked by * (where P <0.05). Full size image Relative to home cage, context exposures robustly induced arc in CA3 neurons (range 38.1–58.0%; Fig. 1d and Supplementary Fig. S4 ), consistent with previous experiments showing that spatial exploration reliably increases arc mRNA [8] . Overall levels of cytoplasmic and nuclear arc were similar in VEH- and TMZ-treated mice ( Supplementary Table S1 ), indicating that TMZ treatment did not alter the likelihood of arc induction. However, the degree of overlap between populations of CA3 neurons activated by the first versus second context exposure varied across groups and across conditions ( Fig. 1d ). In VEH-treated mice, re-exposure to the same context (AA) was more likely to activate the same population of CA3 neurons than exposure to similar (AB) or dissimilar (AC) contexts. Consistent with previous electrophysiological recording and cellular imaging experiments in rats [3] , [4] , [5] , [6] , these data indicate that different contexts are represented, in part, by distinct populations of CA3 neurons (or a population code) (although the magnitude of separation is less than in rats [6] ). In contrast, TMZ treatment impaired this population-based coding of different contexts. Activation of the same population of CA3 neurons was equally likely in the AA and AB conditions (but reduced in the AC condition) ( Fig. 1d ). Therefore, these data indicate that reducing DG neurogenesis impairs population coding of similar, but not dissimilar (or novel), contexts by downstream CA3 neurons. In the TMZ-treated mice, the population of CA3 neurons activated by the second context exposure was larger than that activated by the first context exposure ( Fig. 1f , Supplementary Table S2 ). In an additional experiment, where we reversed the order of context presentation (BA rather than AB; Supplementary Fig. S5 ), we found a similarly expanded population of CA3 neurons active on the second exposure in TMZ-treated mice ( Fig. 1f , Supplementary Table S1 ). Therefore, this suggests that increased overlap of population codes in TMZ-treated mice is primarily driven by an expansion of the population of cells activated by the second exposure. Genetic reduction of neurogenesis impairs population coding We next used a genetic approach to reduce adult neurogenesis. To do this, we used transgenic mice in which a modified HSV-tk gene is expressed from the nestin promoter/enhancer (TK + mice) [10] . In these mice, the administration of ganciclovir (GAN), a nucleoside analogue, ablates only the dividing cells expressing tk. Accordingly, adult TK + mice and their WT littermate controls were treated with GAN for 4 weeks, and then population coding of similar contexts by CA3 neurons was evaluated as above. Neurogenesis was reduced in TK + mice treated with GAN (reduced number of cells expressing Ki67 and NeuroD; Fig. 2a ), without any obvious change in general health or behaviour ( Supplementary Fig. S6 ). As before, in WT mice re-exposure to the same context (AA) was more likely to activate the same population of CA3 neurons than exposure to similar (AB) contexts. In contrast, activation of the same population of CA3 neurons was equivalently likely in the AA and AB conditions in the GAN-treated TK + mice ( Fig. 2c–e and Supplementary Fig. S7 ). Therefore, although chemical and genetic reduction of adult neurogenesis differed in magnitude, they produced equivalent disruption of population coding. This suggests that CA3 population coding of similar context is highly sensitive to fluctuations in neurogenesis, with even modest reductions being sufficient to abolish population-based discrimination of similar contexts. 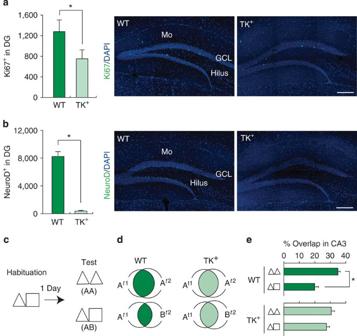Figure 2: Genetic suppression of adult neurogenesis impairs hippocampal coding of similar contexts. (a) Ki67+and (b) NeuroD+staining was reduced in GAN-treated TK+compared with WT mice ((Ki67:t15=3.20,P<0.01; WT,n=9, TK+,n=8); (NeuroD:t9=10.30,P<0.001; WT,n=6, TK+,n=5)). Scale, 200 μm. Mo, molecular layer, GCL, granule cell layer. (c) Experimental design. Mice were habituated to contexts A and B, and then either tested in context A consecutively (AA; WT,n=4, TK+,n=4) or context A then context B (AB; WT,n=5, TK+,n=4). (d) Venn diagrams indicating populations of CA3 cells activated either by first (t1), second (t2) or both (overlap, shaded) context exposures, as reflected byarcexpression. (e) Percent of CA3 cells activated by both context exposures in GAN-treated WT versus TK+mice (Genotype × Context interaction,F1,13=8.28,P<0.05; WTAAversus WTAB,t7=4.91,P<0.001). In these graphs, error bars represent s.e.m., and significantly different contrasts are marked by * (whereP<0.05). Figure 2: Genetic suppression of adult neurogenesis impairs hippocampal coding of similar contexts. ( a ) Ki67 + and ( b ) NeuroD + staining was reduced in GAN-treated TK + compared with WT mice ((Ki67: t 15 =3.20, P <0.01; WT, n =9, TK + , n =8); (NeuroD: t 9 =10.30, P <0.001; WT, n =6, TK + , n =5)). Scale, 200 μm. Mo, molecular layer, GCL, granule cell layer. ( c ) Experimental design. Mice were habituated to contexts A and B, and then either tested in context A consecutively (AA; WT, n =4, TK + , n =4) or context A then context B (AB; WT, n =5, TK + , n =4). ( d ) Venn diagrams indicating populations of CA3 cells activated either by first ( t 1 ), second ( t 2 ) or both (overlap, shaded) context exposures, as reflected by arc expression. ( e ) Percent of CA3 cells activated by both context exposures in GAN-treated WT versus TK + mice (Genotype × Context interaction, F 1,13 =8.28, P <0.05; WT AA versus WT AB , t 7 =4.91, P <0.001). In these graphs, error bars represent s.e.m., and significantly different contrasts are marked by * (where P <0.05). Full size image Neurogenesis regulates behavioural context discrimination Using the same context manipulations as above, we confirmed that suppression of adult neurogenesis produces parallel behavioural effects [11] , [12] . To do this, we used a fear-learning task to evaluate discrimination between similar or dissimilar contexts. In the first experiment, VEH- and TMZ-treated WT mice were pre-exposed to two similar contexts, located in the same room. The next day they were placed in one of the contexts and shocked immediately, and then conditioned freezing was assessed in both the shock-paired versus shock-unpaired context ( Fig. 3a ). During testing, both VEH- and TMZ-treated mice froze more in the context paired with shock versus the no shock context ( Fig. 3b ). However, the degree of discrimination differed, with TMZ-treated mice exhibiting reduced levels of discrimination of these similar contexts compared with VEH-treated controls ( Fig. 3c ). Importantly, discrimination depended upon context pre-exposure, as both VEH- and TMZ-treated mice that were not pre-exposed exhibited low and equivalent levels of freezing in either context when tested ( Supplementary Fig. S8 ). In contrast, discrimination of dissimilar contexts was not affected by chemical reduction of adult neurogenesis ( Fig. 3d ). During testing, both VEH- and TMZ-treated mice froze more in the context paired with shock versus the no shock context ( Fig. 3e ), and the degree of discrimination of these dissimilar contexts did not differ ( Fig. 3f ). We found similar impairments in behavioural discrimination following genetic reduction of adult neurogenesis in TK + mice ( Supplementary Fig. S9 ). Therefore, consistent with our finding that suppression of adult neurogenesis in DG impaired population coding of contexts A and B, these results indicate that suppression of adult neurogenesis impaired behavioural discrimination of these same contexts. We note that freezing levels in the context paired with shock were generally reduced following suppression of adult neurogenesis. Using standard contextual fear-conditioning paradigms, previous studies have sometimes found deficits following suppression of adult neurogenesis (for example, [13] , [14] ), whereas others have not (for example, [14] , [15] ). The present results therefore additionally indicate that prior experience in the contexts may modulate the impact of neurogenesis suppression on contextual learning. 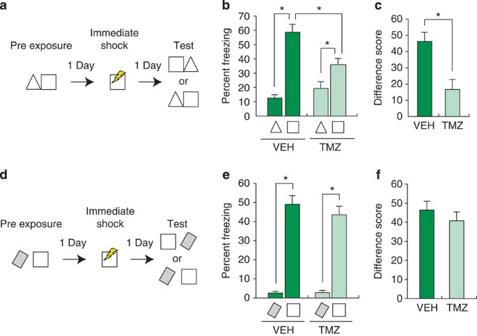Figure 3: Chemical suppression of adult neurogenesis impairs behavioural discrimination of similar contexts. (a) Experimental design (similar contexts). Mice were preexposed to contexts A (triangle) and B (square). The following day they received an immediate shock in context B, and then 24 h later freezing was assessed in contexts A and B. (b) During the test, both VEH-treated (n=11) and TMZ-treated (n=12) mice froze more in context B versus A (Context main effect,F1,21=56.83,P<0.001). (c) However, discrimination (freezingA−freezingB) was reduced in TMZ-treated mice (unpairedt-test,t21=3.54,P<0.01). (d) Experimental design (dissimilar contexts). Mice were preexposed to a rectangular context (located in a different room) and the square context. The following day they received an immediate shock in the square context, and then 24 h later freezing was assessed in the square versus rectangular contexts. (e) During the test, both VEH-treated (n=12) and TMZ-treated (n=12) mice froze more in the square versus rectangular context (Context main effect,F1,44=165.06,P<0.001). (f) Discrimination (freezingA−freezingB) was similar in TMZ-treated mice (unpairedt-test,t22=0.82,P>0.05). In these graphs, error bars represent s.e.m., and significantly different contrasts are marked by * (whereP<0.05). Figure 3: Chemical suppression of adult neurogenesis impairs behavioural discrimination of similar contexts. ( a ) Experimental design (similar contexts). Mice were preexposed to contexts A (triangle) and B (square). The following day they received an immediate shock in context B, and then 24 h later freezing was assessed in contexts A and B. ( b ) During the test, both VEH-treated ( n =11) and TMZ-treated ( n =12) mice froze more in context B versus A (Context main effect, F 1,21 =56.83, P <0.001). ( c ) However, discrimination (freezing A −freezing B ) was reduced in TMZ-treated mice (unpaired t -test, t 21 =3.54, P <0.01). ( d ) Experimental design (dissimilar contexts). Mice were preexposed to a rectangular context (located in a different room) and the square context. The following day they received an immediate shock in the square context, and then 24 h later freezing was assessed in the square versus rectangular contexts. ( e ) During the test, both VEH-treated ( n =12) and TMZ-treated ( n =12) mice froze more in the square versus rectangular context (Context main effect, F 1,44 =165.06, P <0.001). ( f ) Discrimination (freezing A −freezing B ) was similar in TMZ-treated mice (unpaired t -test, t 22 =0.82, P >0.05). In these graphs, error bars represent s.e.m., and significantly different contrasts are marked by * (where P <0.05). Full size image Pattern separation is a neurocomputational construct, referring to the process of transforming similar (overlapping) representations into distinct, orthogonalized codes [2] , [16] . Using a cellular imaging approach, we found that different contexts were coded by distinct populations of neurons in the hippocampal CA3 region in intact WT mice, consistent with the idea that DG-CA3 circuits disambiguate representations of similar contexts [3] , [4] , [5] , [6] . In contrast, both chemical and genetic suppression of adult neurogenesis in DG impaired this CA3 population coding of contexts. In particular, we found that adult neurogenesis suppression impaired coding of similar (but not dissimilar) contexts, consistent with the idea that reducing neurogenesis would hinder resolution of small (but not larger) differences in mnemonic input. This impaired population coding was reflected by an increase in the number of cells that were co-activated by both contexts. However, it appeared that this increased overlap was associated with an expansion of the population of CA3 neurons activated by the second context exposure rather than a decrease in segregation of populations of CA3 neurons activated by each context. The latter is the process of orthogonalization that has been historically associated with pattern separation in the literature, and therefore our results indicate that experimental reduction of neurogenesis leads to less distinct population codes of similar contexts, but not necessarily via a reduction in orthogonalization. In parallel, we found chemical or genetic reduction of adult neurogenesis impaired behavioural discrimination of the same contexts. These results are consistent with recent findings that reducing neurogenesis impedes spatial discrimination [11] , [12] , [17] , whereas enhancing neurogenesis promotes spatial discrimination [11] , [18] , and provide an essential link between the effects of manipulating levels of adult neurogenesis on behaviour and changes in information processing in hippocampal networks. New neurons have been proposed to facilitate population coding of contexts either by directly promoting remapping in place cells in CA3 or indirectly by activating dentate inhibitory neurons that lead to increased sparsification of DG codes that then feed forward into CA3 (ref. 19 , 20 ). Our data indicate that new neurons facilitate disambiguation of contexts by regulating activity of CA3 neurons, and thereby reducing overlap in population codes. Mice In these experiments we used two lines of mice. First, in the chemical suppression of adult neurogenesis experiments we used male WT offspring from a cross between C57Bl/6NTacfBr (C57B6) and 129Svev (129) mice (Taconic). Second, in genetic suppression of adult neurogenesis experiments we used transgenic mice expressing a modified HSV-tk under control of the nestin promoter (TK + mice) [10] . These mice were maintained on a C57B6 background (>8 crosses), and experimental mice were generated by crossing TK + mice with C57B6 WT mice (for arc fluorescent in situ hybridization experiments) or with 129 WT mice (for fear conditioning experiments). Male and female TK + and WT littermates were used in experiments. All mice were bred in our colony at The Hospital for Sick Children, maintained on a 12 h light/dark cycle with free access to food and water. Behavioural procedures were conducted during the light phase of the cycle, blind to genotype of the mouse and according to protocols approved by the Animal Care Committee at The Hospital for Sick Children. Chemical suppression of adult neurogenesis Starting at 6 weeks of age, WT mice were treated with the DNA-alkylating agent TMZ (Sigma) for 4 weeks. We used an established injection protocol that has previously been shown to reliably suppress neurogenesis in adult mice [9] . During each of the 4 weeks of treatment, mice received daily injections of TMZ (25 mg kg −1 intraperitoneally) for 3 consecutive days, followed by 4 days of no injections. TMZ was dissolved in 10% dimethyl sulfoxide. The VEH group received injections of 10% dimethyl sulfoxide. Genetic suppression of adult neurogenesis For arc in situ hybridization experiments, TK + mice and their WT littermate controls were treated with GAN (200 mg kg −1 per day, Cytovene-IV, Roche Pharmaceuticals) delivered via osmotic minipumps (model 2002, Alzet). Pumps were implanted subcutaneously at 8 weeks of age as previously described [10] . For behavioural experiments, GAN was mixed into powdered chow (0.08%, ~70 mg kg −1 per day) (ref. 21 ), and TK + mice and their WT littermate controls had ad lib access to the chow in their home cage for 28 days, starting at 8 weeks of age. Immunohistochemistry Following testing, mice were decapitated and brains were frozen on dry ice. Coronal sections (20 μm) were cut using a cryostat. All sections were treated with 1% hydrogen peroxidase. Sections were then incubated overnight with the primary antibodies (anti-Ki67 (1/100; Chemicon) or anti-NeuroD (1/150; Santa Cruz)) at 4 °C and then for 60 min at 20 °C with horseradish peroxidase (HRP)-conjugated secondary antibodies (1:300; Jackson Immuno-research, PA), and developed with an Alexa 488-conjugated tyramide amplification system (PerkinElmer) ( [8] , [22] See refs 8,22). Sections were mounted on slides with Permafluor anti-fade medium, and counter-stained with Hoechst 33258 to mark nuclei. Ki67 + and NeuroD + cells were quantified using an epifluorescent microscope (Nikon Eclipse 80i) with × 40 objective. To generate cell counts we used 1/6 systematic section sampling fractions covering the entire anterior–posterior extent of the DG. arc fluorescent in situ hybridization Coronal sections (20 μm) were cut and thaw-mounted on slides, such that each slide contained sections from different treatment conditions (to maximize relevant between-group comparisons within each slide). Digoxigenin (DIG)-labelled antisense and sense riboprobes for arc mRNA were generated using a commercial transcription kit (MaxiScript, Ambion) and RNA labelling mix (Roche Diagnostics) from a plasmid encoding arc open reading frame. arc antisense riboprobe was detected with an anti-DIG antibody conjugated with HRP FAB fragments (1/300; JacksonImmunoResearch) and developed with an Alexa 488-conjugated tyramide amplification system (PerkinElmer) ( [8] , [22] See refs 8,22). Briefly, sections were fixed with 4% paraformaldehyde fixation buffer, washed in 2 × 0.3 M sodium chloride and 0.03 M SSC, treated with 0.5% acetic anhydride/1.5% triethanolamine, and 50% methanol/50% acetone before being incubated in hybridization buffer (with 50% formamide, 5 × SSC, 0.1 mg ml −1 yeast transfer RNA, 0.1% Tween-20 and 50 mg ml −1 Heparin) for 30 min at 20 °C. Sections were incubated with arc riboprobe (1 ng μl −1 in hybridization buffer) at 56 °C overnight. Twenty-four hours later, sections were treated sequentially with RNaseA (10 μg ml −1 in 2 × SSC at 37 °C for 30 min), followed by two washes in 0.5 × SSC at 56 °C. Sections were then treated with hydrogen peroxide (1% for 30 min), blocking reagent (Roche Diagnostics) with goat serum (4%) (30 min) and incubated with an anti-DIG HRP-conjugated antibody (described above) in blocking solution for 2 h at 20 °C. Tyramide amplification was performed for 30 min at 20 °C. Nuclei were visualized with Hoechst 33258 (Sigma) counterstain. Images were captured using a confocal microscope (Zeiss LSM 710 equipped argon diode laser). Images were acquired using a X40 oil-immersion lens and z-sectioned in 1 μm thick optical sections. Images were collected from CA3 (AP: ~−2.0 mm from bregma) [23] , and every third section was analysed. Microscope settings (pinhole, gain and contrast) were kept constant for all images on a given slide. Localization of arc signal was analysed using Image-Pro PLUS software (MediaCybernetics). Small, bright uniformly DAPI stained nuclei (roughly 5 μm in diameter) from putative glial cells were not counted. All other whole nuclei cells (putative neurons) in the field of view within the CA3 region were counted. Nuclear arc was defined as focal arc puncta in the nucleus whereas cytoplasmic arc was defined as arc -positive dots surrounding the nucleus. Nuclei were only considered if they could be discerned in their entirety through the z-sectioned images. Manual cell counts were performed by an observer unaware of the treatment condition. Two to four sections were analysed per mouse, and the number of CA3 cells having intranuclear foci and/or cytoplasmic signals of arc mRNA were counted. Contexts The three contexts (A (triangular), B (square) and C (rectangular); Supplementary Fig. S2 ) used in these experiments have been previously described [24] . Contexts A and B were located in the same room. Context C was located in a different room. Arc in situ fluorescent hybridization experiments Before behavioural testing, mice were handled daily for 2 min each across 4 days. Behavioural testing was conducted on 2 consecutive days, starting immediately following completion of the 4-week TMZ/GAN treatment. On the first day (habituation), mouse home cages were transported from the vivarium to a quiet, holding area in the behavioural lab. After 1 hour acclimation, mice were placed in context A for 5 min, and then returned to their home cage. Approximately 1 h later, mice were placed in context B for 5 min and then returned to their home cage and taken back to the vivarium. The following day (testing), mice were acclimated for 1 h, and then placed in context A for 5 min. They were immediately returned to their home cage, and then 20 min later placed in context A (AA condition), context B (AB condition) or context C (AC condition) for 5 min. Additional groups of VEH- and TMZ-treated mice were treated identically, but tested in B then A (BA condition). Immediately following this, mice were killed by decapitation and brains were removed and frozen on dry ice. Mice in the home cage group were decapitated in the vivarium. Fear conditioning experiments To evaluate whether suppression of adult neurogenesis impairs context discrimination we adapted a fear-conditioning paradigm [25] , [26] . During the last 4 days of TMZ/VEH (chemical suppression) or GAN (genetic suppression) treatments, mice were handled daily for 2 min each. Behavioural testing was conducted over 3 consecutive days, starting following completion of TMZ treatment/handling. On the first day (preexposure), mouse home cages were transported from the vivarium to a quiet, holding area in the behavioural lab. After 1 hour acclimation, mice were placed in context A for 5 min, and then returned to their home cage. Approximately 1 h later, mice were placed in context B for 5 min and then returned to their home cage and taken back to the vivarium. The following day, mice were placed in context B, where they received an immediate shock (1.0 mA, 2 s duration). They remained in the context for an additional minute and were then taken back to the vivarium. The following day, mice were tested in both context A and context B, in a counter-balanced order. Tests were 5 min in duration, and spaced 1 h apart. To test whether context discrimination depended on context preexposure, additional groups of mice were treated as above, but not preexposed to the contexts. To test whether chemical reduction of neurogenesis impaired discrimination of dissimilar contexts, we conducted an additional experiment. All procedures were identical, except that the square and rectangular (located in different room) contexts were used. During the preexposure, training and testing phases, mouse behaviour was monitored via four overhead cameras. Freezing behaviour was assessed using an automated scoring system (Actimetrics, Wilmette, IL), which digitized the video signal at 4 Hz and compared movement frame by frame to determine the amount of freezing. Statistical analyses Effects of manipulating adult neurogenesis on arc induction and behaviour were evaluated by analysis of variance followed by t -tests or Tukey post-hoc tests where appropriate. In graphs, data are presented as mean±s.e.m. How to cite this article: Niibori, Y. et al . Suppression of adult neurogenesis impairs population coding of similar contexts in hippocampal CA3 region. Nat. Commun. 3:1253 doi: 10.1038/ncomms2261 (2012).